Unravelling cerebellar pathways with high temporal precision targeting motor and extensive sensory and parietal networks Increasing evidence has implicated the cerebellum in providing forward models of motor plants predicting the sensory consequences of actions. Assuming that cerebellar input to the cerebral cortex contributes to the cerebro-cortical processing by adding forward model signals, we would expect to find projections emphasising motor and sensory cortical areas. However, this expectation is only partially met by studies of cerebello–cerebral connections. Here we show that by electrically stimulating the cerebellar output and imaging responses with functional magnetic resonance imaging, evoked blood oxygen level-dependant activity is observed not only in the classical cerebellar projection target, the primary motor cortex, but also in a number of additional areas in insular, parietal and occipital cortex, including sensory cortical representations. Further probing of the responses reveals a projection system that has been optimized to mediate fast and temporarily precise information. In conclusion, both the topography of the stimulation effects and its emphasis on temporal precision are in full accordance with the concept of cerebellar forward model information modulating cerebro-cortical processing. Despite the wealth of evidence that the cerebellum has a role in motor control, a number of observations implicate that the cerebellum is also involved in sensory functions. The most conspicuous example is probably the extraordinarily enlarged cerebellum in weakly electric fish, which was soon associated with an involvement in (electro-) sensation [1] . A model by Kawato [2] proposes that the cerebellum performs as a forward model to provide predictions of the sensory feedback. Sensory predictions could facilitate the fine-tuning of motor acts and may also help to deal with the perceptual consequences of actions [3] . The forward model hypothesis may therefore provide a unifying computational basis that could account for the well-established role of the cerebellum in motor control as well as for its role in perception [4] , [5] , [6] . Forward models are crucial to short-cut the long feedback delays (100–200 ms) that occur during motor actions. Recent studies [7] have shown that most information is contained within the first 10–20 ms of a sensory event. High temporal precision would therefore be an important additional requirement of a forward sensory predictor. The cerebellar microcircuit is ideally suited to provide for such precision. The majority of neurons in the cerebellum (and in the whole brain [8] ) are the granule cells. Via their parallel fibres, these cells provide a short-lived excitatory feed-forward computation of the order of milliseconds [9] . On the basis of the theory that the cerebellum is a sensory predictor, we would expect the cerebellar output to show high temporal precision and to emphasize motor and sensory targets. However, studies of cerebello–cerebral connections using conventional anatomical techniques only partially meet this requirement. We decided to readdress the structure of cerebello–cerebral connections by using a novel technique that enabled us to delineate a more comprehensive pattern of cerebello–cerebral projections in an individual. Electrical stimulation, combined with functional magnetic resonance imaging (es-fMRI), is an important tool to study the functional properties of the spatially distributed neuronal networks of the brain [10] , [11] , and could be ideally suited to readdress the cerebello–cerebral connections. Our earlier studies in the neocortex showed that the evoked blood oxygen level-dependant (BOLD) responses were due to the stimulation of pyramidal axons [11] . However, irrespective of the stimulation parameters, our striate and extrastriate cortex stimulation did not result in any transsynaptic propagation of the activity within the neocortex. By contrast, electrical stimulation of subcortical structures such as the optical tract revealed transsynaptic propagation of activity through the thalamus to the neocortex [10] . Synaptic pathways therefore show different degrees of efficacy in mediating activity evoked by electrical stimulation. The results presented here confirm that subcortical pathways can propagate electrically induced activity transsynaptically with high efficiency. Furthermore, by stimulating the gateway of the cerebellar output, the deep cerebellar nuclei (DCN), stimulation-induced BOLD activity can be observed not only in the classical cerebellar projection target, the primary motor cortex, but also in a number of additional sensory and parietal areas. This confirms the sensory predictor expectation of the cerebellar output. Responses in this pathway were strongest for very high stimulation frequencies (≥400 Hz) and had short latencies. This points to a projection system that has been optimized to mediate fast and temporarily precise information in full accordance with the concept of cerebellar forward model information modulating cerebro-cortical processing. Characterizing deep cerebellar nuclei connectivity Output from cerebellar–cortex converges on the deep cerebellar nuclei (DCN), which in turn, maintains projections to a number of extracerebellar targets. By electrically stimulating the DCN or, alternatively, the fibre bundles arising from the DCN in the superior cerebellar peduncle (SCP) in 22 experimental sessions involving four monkeys, we acquired stimulation-evoked BOLD signals with fMRI. We also performed electrophysiological recordings of stimulation-induced field potentials in cerebral cortex to examine the temporal characteristics of the cerebellar influence on cerebral cortex in more detail. To prevent muscle activation due to DCN stimulation and BOLD activity secondary to overt stimulation-induced motor responses, all experiments were carried out under general anaesthesia and muscle relaxation. On the basis of earlier anatomical studies, we anticipated that the bulk of stimulation-induced BOLD responses in cerebral cortex would be located in primary motor cortex through the main cerebellar thalamic nuclei (VPLo, X, VLc [12] ). However, we consistently observed that stimulation of the DCN evoked BOLD responses in much larger cerebro-cortical networks ( Fig. 1a,b; Supplementary Fig. S1 ). BOLD responses were largely confined to the grey matter. The observed stimulation patterns were robust in individual experiments and were obtained in all monkeys. Responses were typically evoked already by the first stimulus train ( Fig. 1c ). Surprisingly, cerebro-cortical stimulation-evoked BOLD responses were not confined to the contralateral hemisphere. Instead, we consistently observed bilateral and largely symmetrical cerebro-cortical BOLD responses. This is at variance with prevailing anatomical evidence that most DCN output fibres terminate in the contralateral thalamic nuclei [12] . 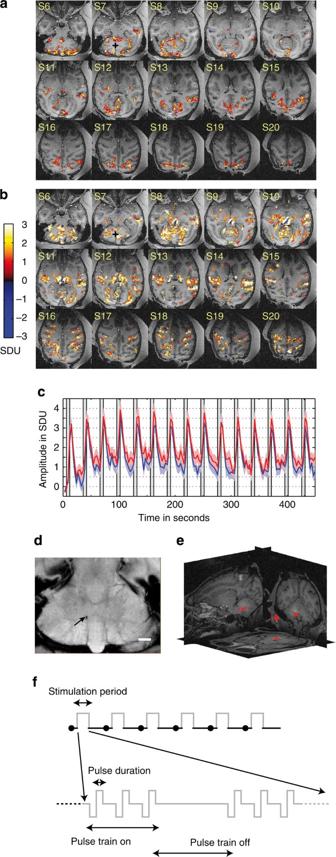Figure 1: Electrical stimulation of the DCN elicits BOLD activation in cortical and subcortical regions. (a,b) Consecutive horizontal sections are shown with overlaid statistical maps for two different current intensities, 63 μA (a) and 250 μA (b). (c) Example of the time course of BOLD responses following electrical stimulation of the DCN (Experiment A05id1). Time course of thalamus ROI on the contralateral side in respect to the electrode location (mean and s.e. of the mean; 75 repetitions) is marked in red (ipsilateral in blue). Grey bars indicate periods of stimulation. (d) Electrode tip location of experiment shown in (a) and (b). Scale bar is 5 mm. The overlay on 3D model derived from histological sections locates stimulation site within NIP. (e) Summary of all DCN electrode tip locations. (f) Beginning of stimulation trials are each noted with a black dot and typically consisted of a 9-s resting period (black line) followed by 6 s-stimulation (grey line) and 15 s of resting (black line). During the stimulation period, pulse trains consisting of biphasic charge-balanced pulses were applied. Single-pulse duration was typically 200 μs per phase. These pulses were applied in trains (bursts) in periods termed pulse train on with interspersed pauses termed pulse train off. Typically, we applied pulses at 400 Hz for a 200 ms (pulse train on) period interspersed with a 400 ms pulse train off period. Figure 1: Electrical stimulation of the DCN elicits BOLD activation in cortical and subcortical regions. ( a,b ) Consecutive horizontal sections are shown with overlaid statistical maps for two different current intensities, 63 μA ( a ) and 250 μA ( b ). ( c ) Example of the time course of BOLD responses following electrical stimulation of the DCN (Experiment A05id1). Time course of thalamus ROI on the contralateral side in respect to the electrode location (mean and s.e. of the mean; 75 repetitions) is marked in red (ipsilateral in blue). Grey bars indicate periods of stimulation. ( d ) Electrode tip location of experiment shown in ( a ) and ( b ). Scale bar is 5 mm. The overlay on 3D model derived from histological sections locates stimulation site within NIP. ( e ) Summary of all DCN electrode tip locations. ( f ) Beginning of stimulation trials are each noted with a black dot and typically consisted of a 9-s resting period (black line) followed by 6 s-stimulation (grey line) and 15 s of resting (black line). During the stimulation period, pulse trains consisting of biphasic charge-balanced pulses were applied. Single-pulse duration was typically 200 μs per phase. These pulses were applied in trains (bursts) in periods termed pulse train on with interspersed pauses termed pulse train off. Typically, we applied pulses at 400 Hz for a 200 ms (pulse train on) period interspersed with a 400 ms pulse train off period. Full size image One might argue that this multifocal pattern of cerebral responses was owing to the fact that the stimulation current spread across the midline, affecting DCN output on the opposite side as well as neighbouring neurons and fibres that did not belong to the cerebello–cerebral projection. To address this concern, we routinely verified electrode tip location with MRI ( Fig. 1d,e ) and mapped the location, in one case, with additional histological examination and three-dimensional (3D)-reconstruction of the DCN (monkey A06; Supplementary Fig. S2 ). We also estimated the critical current spread by calculating the voltage gradient and by validating our results with previous experimental results. In Supplementary Fig. S2F , we plotted the critical region surrounding the DCN electrode positions and ascertained that it was largely limited to the cerebellum and did not extend to the brain stem. Extended multifocal bilateral cerebro-cortical response patterns could be evoked with currents as low as 63 μA. Stimulation trials typically consisted of a 9-s resting period ( Fig. 1f ) followed by 6 s of stimulation and 15 s of resting. Biphasic charge-balanced pulses were applied during the stimulation period. Pulses were applied in bursts of 200 ms length (pulse train on) interspersed with pauses of 400 ms (pulse train off). Increasing stimulation strength from 63 to 250 μA ( Fig. 1a,b ) led to an increase in the number of patches, without changing the balance between ipsilateral and contralateral response and without significantly changing the boundaries of the area activated. We also tested a bipolar electrode instead of standard monopolar electrodes in an attempt to reduce current spread ( Supplementary Figs S3 and S4 ). However, this type of electrode yielded very similar multifocal bilateral responses as evoked by monopolar electrodes, although the estimated excited tissue volume was reduced from 11.5 to 1.5 mm 3 (with 100 μA stimulation; see Supplementary Fig. S4A ). Fibres originating from the DCN pass to the opposite side at the level of the SCP. In experiments in which the stimulation electrode was located in the SCP, it may have activated fibres that already crossed sides as well as fibres that would not cross until later, thereby giving rise to bilateral cerebro-cortical responses. However, bilateral responses were not confined to SCP stimulations. In fact, stimulation of the fastigial nucleus, the most medial part of the DCN, also gave rise to bilateral responses ( Supplementary Fig. S1A ), a finding that seems to be at odds with the textbook view of a strictly contralateral projection from the DCN. However, it is well established that fastigial neurons target thalamic regions bilaterally [13] , which may also explain the bilaterality of evoked cerebro-cortical responses in this case. We also obtained bilateral cerebro-cortical stimulation responses after stimulating the posterior interposed nucleus (NIP). However, with respect to this nucleus, it is not known as to whether the projection is strictly contralateral. Mapping subcortical and cortical hotspots To unravel the pathways underlying the multifocal cerebro-cortical responses in more detail, we used the atlas of Olszewski [14] to carefully map the activation patterns within the thalamus, the likely mediator of the signals emerging from the DCN/SCP. In Fig. 2 and Supplementary Figs S5 and S6 , the activation hotspots (averages of 5 and 7 experiments, respectively, for two monkeys) are shown mapped on the appropriate atlas sections. Hotspots were located bilaterally in VPLo (Nucleus ventroposterior lateral pars oralis of the thalamus)/VLc (ventral lateral nucleus, pars caudalis of the thalamus) [14] , CL (Centralis lateralis)/CN.Md (Nucleus centrum medianum), CL bordering MDdc (mediodorsal thalamic nucleus pars densocellularis), LP (lateral posterior nucleus), Pul.m (nucleus pulvinaris pars medialis), MD.dc and SG (Suprageniculate nucleus). Very little activation was observed in VA (ventral anterior thalamic nucleus) and in the MD (mediodorsal thalamic nucleus) proper. As mentioned earlier, previous work based on conventional anatomical tracing techniques has suggested that the numerically major output of the DCN is destined to specific contralateral thalamic subnuclei VPLo, X (Nucleus X of the thalamus) and VLc, which in turn project to the motor cortex [12] . In addition, a numerically less prominent projection to the contralateral intralaminar nucleus has been delineated [15] , [16] . Hence, one scenario able to explain our discovery of multiple regions of activation within the contralateral cerebro-cortical hemisphere is that there are additional pathways involving other thalamic nuclei such as the intralaminar nuclei. In fact, in accordance with this scenario, earlier studies in the cat using electrical stimulation of the DCN and local field potential (LFP) recordings [17] showed that the DCN projects to the cerebral cortex via at least two high-frequency thalamic channels: via the VA/VL (ventrolateral thalamic nucleus) which correspond to monkey VPLo, X, VLc and via a thalamic region called ventromedial thalamic nucleus, which, in turn, projects to wide-spread cortical regions [17] . In summary, mapping the BOLD responses in the thalamic nuclei revealed that in addition to the classic cerebellar recipient nuclei, additional thalamic nuclei such as the intralaminar thalamic nuclei were also involved. Parts of these nuclei have been suggested to carry an efference copy signal [18] . 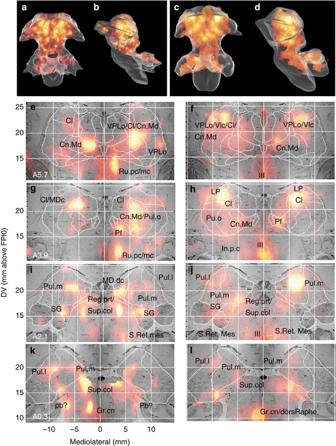Figure 2: Identifying subcortical hot spots mediating multifocal cortical responses. (a–d) 3D semi-transparant view of brain stem and diencephalon. Activation maps are shown as colour-coded maximum intensity projections. (Panelsaandc) show the posterior view, whereas in (b) and (d), a lateral view is shown for two monkeys (a,b, A05 andc, d, A07). (e–l) Average responses for two monkeys of activated regions superimposed on the Olszewski thalamus atlas for the macaque14. Monkey A05 (left panelse,g,i,k, averages of 5 experiments) and A07 (right panelsf,h,j,l, averages of 7 experiments). Shown are the coronal sections at different anterior–posterior positions 0.3, 2.1, 3.9, 5.7 (with 0 corresponding to the interaural line). White grid lines are 5 mm apart (dorso-ventral (DV): 10,15, 20 and 25 mm above the interaural-Frankfurt plane (FPl)). Activation can be observed in classical cerebellar-receiving thalamus regions (VPLo, VLc), as well as in additional regions Cn.Md, Cl, LP and Nucleus pulvinaris pars oralis (Pul.o). Pcn, nucleus paracentralis; Pf, nucleus parafascicularis; Reg. Prt, regio pretectalis; Ru, nucleus ruber; S. Ret. Mes, substantia reticularis mesencephali; Gr.cn, griseum centralis; In.p.c, nucleus interstitialis posterior commisure. Figure 2: Identifying subcortical hot spots mediating multifocal cortical responses. ( a–d ) 3D semi-transparant view of brain stem and diencephalon. Activation maps are shown as colour-coded maximum intensity projections. (Panels a and c ) show the posterior view, whereas in ( b ) and ( d ), a lateral view is shown for two monkeys ( a , b , A05 and c, d , A07). ( e–l ) Average responses for two monkeys of activated regions superimposed on the Olszewski thalamus atlas for the macaque [14] . Monkey A05 (left panels e , g , i , k , averages of 5 experiments) and A07 (right panels f , h , j , l , averages of 7 experiments). Shown are the coronal sections at different anterior–posterior positions 0.3, 2.1, 3.9, 5.7 (with 0 corresponding to the interaural line). White grid lines are 5 mm apart (dorso-ventral (DV): 10,15, 20 and 25 mm above the interaural-Frankfurt plane (FPl)). Activation can be observed in classical cerebellar-receiving thalamus regions (VPLo, VLc), as well as in additional regions Cn.Md, Cl, LP and Nucleus pulvinaris pars oralis (Pul.o). Pcn, nucleus paracentralis; Pf, nucleus parafascicularis; Reg. Prt, regio pretectalis; Ru, nucleus ruber; S. Ret. Mes, substantia reticularis mesencephali; Gr.cn, griseum centralis; In.p.c, nucleus interstitialis posterior commisure. Full size image Additional projections of the DCN (from the fastigius and interpositus posterior nuclei) could reach wider regions within the thalamus disynaptically via the superior colliculus and periaquaductal grey. Furthermore, subcortical connections via the SG and Pul. m ( Fig. 2 ) could explain the activation of auditory cortex obtained [19] , [20] . In the cat, these nuclei receive direct fastigial [13] and interpositus posterior inputs [21] . To identify the cortical areas that showed BOLD responses, we displayed our activation maps as flat maps, with cortical areas demarcated [22] as in the atlas of the macaque brain by Saleem and Logothetis [23] . 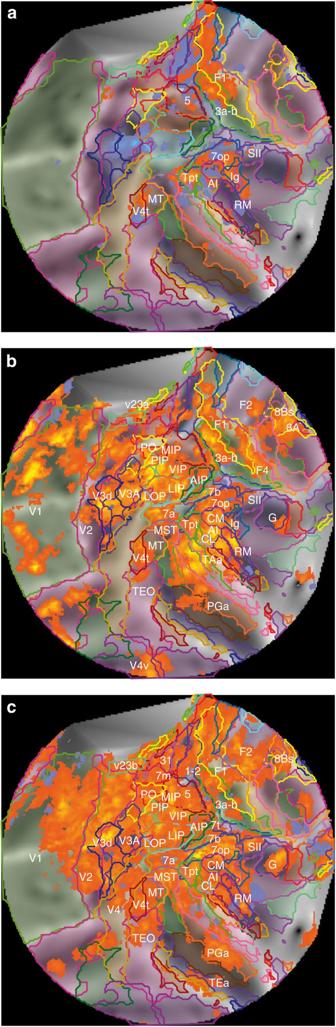Figure 3: Mapping cortical regions on flat maps. In (a–c) the results from stimulating three different sites in three monkeys located in the interpositus nuclei. Different patterns were observed from stimulating NIA (a) compared with NIP (b,c). Stimulation of NIA (a) mainly resulted in responses within the primary motor cortex (F1) and adjoining postcentral gyrus (area3a,b). In addition, parieto-insular and STS responses were evoked. Stimulation of NIP (b,c) gave rise to a complex activation pattern of mainly parieto-occipital cortical areas with a dominance of the dorsal visual stream. Further activation was detected in motor and premotor areas (F1, F2, F4, 8Bs/8A). In (b), activation was also observed in auditory regions (AI, Rm and CL). Figure 3 shows the results following the stimulation of three different sites within the DCN. Stimulation of the anterior interposed nucleus (NIA) ( Fig. 3a ) resulted in extensive positive BOLD responses in both the primary motor cortex (F1) and the postcentral somatosensory cortex (BA 3a–b), in parieto-insular areas 7op, 7b and Ig (granular insula), upper STS (superior temporal sulcus, corresponding to V5/MT) and in area Tpt. Stimulation of a more posterior region within the NIP ( Fig. 3b ) gave rise to a more complex activation pattern. A number of parieto-occipital cortical areas showed BOLD activity with a dominance of responses in areas of the dorsal visual stream, in motor and premotor areas (F1, F2, F4), as well as in areas 8Bs/8A (including area 8Av which corresponds to the frontal eye fields). Interestingly enough, stimulation of the NIP also gave rise to activity in primary auditory area AI as well as in the rostromedial belt regions (Rm) and CL. In a further experiment, we stimulated a different part of the NIP (a more posterior region within NIP, Fig. 3c ). This resulted in BOLD responses in a number of parieto-occipital areas, including peripheral V1 (lower visual field), V2 (lower peripheral visual field extending to an approximate eccentricity of 10° of the visual field) and V3d. Responses were also seen in anterior (AIP), medial (MIP), ventral (VIP), lateral (LIP) intraparietal areas and in parieto-insular areas (7op, 7b and gustatory area G) and in areas in the STS (MT/V5, medial superior temporal area, V4t, temporo-occipital area (TEO) and PGa (parietal area PG-associated area of the STS)). Further examples of stimulation experiments that yielded similarly complex activation patterns are shown in Supplementary Fig. S1 . We add that previous studies employing transneuronal retrograde tracing also showed cerebellar projections to areas AIP and 7b [24] and to LIP and VIP [25] . Figure 3: Mapping cortical regions on flat maps. In ( a–c ) the results from stimulating three different sites in three monkeys located in the interpositus nuclei. Different patterns were observed from stimulating NIA ( a ) compared with NIP ( b , c ). Stimulation of NIA ( a ) mainly resulted in responses within the primary motor cortex (F1) and adjoining postcentral gyrus (area 3a , b ). In addition, parieto-insular and STS responses were evoked. Stimulation of NIP ( b , c ) gave rise to a complex activation pattern of mainly parieto-occipital cortical areas with a dominance of the dorsal visual stream. Further activation was detected in motor and premotor areas (F1, F2, F4, 8Bs/8A). In ( b ), activation was also observed in auditory regions (AI, Rm and CL). Full size image Parametric characterization of the cerebello–cerebral pathway with fMRI One major cerebro-cortical region activated by DCN stimulation were the areas of the dorsal visual pathway in the parieto-occipital lobes, known to process magnocellular input, emphasizing fast and temporarily precise signals [26] . This suggests that also cerebellar input to this region should emphasize fast and temporarily precise signals. This is indeed the case as DCN neurons are known to be able to follow very high-frequency electrical stimulations (up to 800 Hz (ref. 27 )), a feature that correlates with high conduction velocity and precise timing of responses [28] , [29] . In fact, parametric probing supported the anticipated strong dependency of the BOLD responses on high-frequency stimulation as the strength of the BOLD signal grew with frequency up to frequencies of 600 Hz and only then did the signal show signs of saturation ( Fig. 4a,b ; for the SCP, see Supplementary Fig. S7 ). 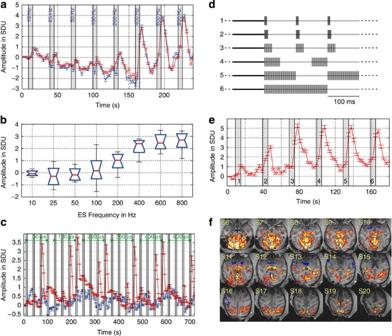Figure 4: Higher frequencies drive polysynaptic DCN-cortical networks. (a) Experiment A051r1 with electrode in SCP bordering NIA. First positive BOLD responses appear at stimulation frequencies of 200 Hz and increase substantially at higher frequencies. Time course of voxels taken from contralateral thalamus. (b) Population results of stimulation frequency effects for contralateral thalamic ROI. Eight different sites were stimulated in two monkeys. Box and whisker plots with upper and lower quartiles inidicated by box lines and the centre line indicates the median. The medians of boxes whose notches do not overlap differ at the 5% level. Whisker length indicates most extreme data that are within the interquartile range of the sample. Data were further analysed with a Kruskal–Wallis one-way ANOVA with stimulation frequency as the dependant variable. The test showed a significant effect (×2=43; df=7,P<0.001;n=8). A Tukey's post-hoc test showed statistical significance of responses with frequencies larger than 400 Hz compared with 100 Hz, as well as between frequencies lower than 100 Hz and 400 Hz. (c) Stimulation of caudal fastigial DCN region (A051b1). 400 Hz (red traces) were effective in yielding strong BOLD responses, whereas 100 Hz (blue) were not. Four different charges were applied at six different pulse durations (50–600 μs): and with currents equivalent to charges of 25, 50, 75 and 100 nC. (d) Stimulation with varying pulse train on periods. (1) Five pulses were delivered within 7ms (600 Hz; repeated every 100ms); (2): 7 pulses within 10 ms (600 Hz; repeated every 100 ms); (3): 10 pulses within 25 ms (400 Hz; repeated every 100 ms); (4): 20 pulses within 50 ms (400 Hz; repeated every 150 ms); (5): 40 pulses within 100 ms (400 Hz; repeated every 200ms); (6): 80 pulses within 200 ms (400 Hz; repeated every 600 ms). In (e), the BOLD amplitude time course of the contralateral thalamic ROI was plotted for the different conditions 1–6 (as ind). (f) Experiment A05NW1 with 10 ms pulse train on (7 pulses at 600 Hz) and 90ms pulse train off (same as in (d) number 2) and current amplitude 250 μA. Error bars indicate standard errors of the mean. Figure 4: Higher frequencies drive polysynaptic DCN-cortical networks. ( a ) Experiment A051r1 with electrode in SCP bordering NIA. First positive BOLD responses appear at stimulation frequencies of 200 Hz and increase substantially at higher frequencies. Time course of voxels taken from contralateral thalamus. ( b ) Population results of stimulation frequency effects for contralateral thalamic ROI. Eight different sites were stimulated in two monkeys. Box and whisker plots with upper and lower quartiles inidicated by box lines and the centre line indicates the median. The medians of boxes whose notches do not overlap differ at the 5% level. Whisker length indicates most extreme data that are within the interquartile range of the sample. Data were further analysed with a Kruskal–Wallis one-way ANOVA with stimulation frequency as the dependant variable. The test showed a significant effect (× 2 =43; df=7, P <0.001; n =8). A Tukey's post-hoc test showed statistical significance of responses with frequencies larger than 400 Hz compared with 100 Hz, as well as between frequencies lower than 100 Hz and 400 Hz. ( c ) Stimulation of caudal fastigial DCN region (A051b1). 400 Hz (red traces) were effective in yielding strong BOLD responses, whereas 100 Hz (blue) were not. Four different charges were applied at six different pulse durations (50–600 μs): and with currents equivalent to charges of 25, 50, 75 and 100 nC. ( d ) Stimulation with varying pulse train on periods. (1) Five pulses were delivered within 7ms (600 Hz; repeated every 100ms); (2): 7 pulses within 10 ms (600 Hz; repeated every 100 ms); (3): 10 pulses within 25 ms (400 Hz; repeated every 100 ms); (4): 20 pulses within 50 ms (400 Hz; repeated every 150 ms); (5): 40 pulses within 100 ms (400 Hz; repeated every 200ms); (6): 80 pulses within 200 ms (400 Hz; repeated every 600 ms). In ( e ), the BOLD amplitude time course of the contralateral thalamic ROI was plotted for the different conditions 1–6 (as in d ). ( f ) Experiment A05NW1 with 10 ms pulse train on (7 pulses at 600 Hz) and 90ms pulse train off (same as in ( d ) number 2) and current amplitude 250 μA. Error bars indicate standard errors of the mean. Full size image By systematically varying stimulation parameters, we further confirmed that the higher stimulation frequency was the relevant parameter for the generation of the robust activation pattern in these polysynaptic networks ( Fig. 4a,b ). Unlike in cerebral cortex [10] , [11] , where electrical pulses at frequencies as low as 100 Hz evoke reliable BOLD responses (amplitudes of 3 standard deviation units (SDU), Fig. 5 in ref. 10 ), stimulation of the DCN yielded robust responses mainly at frequencies of and above 400 Hz ( Fig. 4b ; Supplementary Fig. S8 ), which only saturated at 600 Hz. A statistical test (a one-way ANOVA ( F =11.18; P <0.001; n =8) and the multiple comparison procedure based on Tukey's tests showed significant differences between the responses at 50 and 400 Hz. The BOLD amplitudes at 50 and 200 Hz were not significantly different. The importance of frequency was further substantiated by examining the influence of current amplitude and pulse duration ( Fig. 4c ). In this example, stimulation with 100 Hz yielded weak (<1 SDU) BOLD responses in the thalamic nuclei independent of the current amplitudes or pulse durations used. On the other hand, altering the stimulation frequency to 400 Hz yielded strong responses with charges above 75nC. 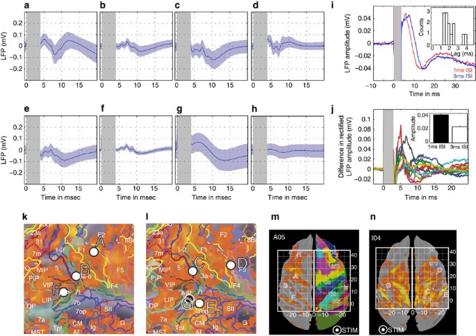Figure 5: LFP and BOLD responses following stimulation of the cerebellar output. (a–h) LFPs following a 4-pulse burst are shown. Stimulation periods ina–jare indicated by grey rectangles. Sites from which the recordings was obtained are plotted inkandlonto flatmaps for the two monkeys (A05, I04). (a) contralateral precentral gyrus (mapped to F1); (b) contralateral postcentral gyrus (mapped to 1-2); (c) contralateral postcentral gyrus (mapped to 1-2 bordering BA5); (d) contralateral precentral gyrus (mapped to F4); (e) contralateral postcentral gyrus (mapped to border of 7b and 7op); (f) contralateral intraparital sulcus (mapped to AIP); (g) ipsilateral intraparital sulcus (mapped to border AIP/7t/7a); (h) prefrontal cortex (mapped to BA 46d). A number of traces show high-frequency responses following the stimulus. Contralateral recording sites show greatest deflections at 5–12 ms, with the earliest appearing 2–4 ms (a–f). Ipsilateral responses show greatest immediate responses at 5–7 ms (g). (i,j) DCN stimulation with double pulses. In I, results are shown from recording site G (ipsilateral to DCN stimulation side, mapped to border AIP/7t/7a). In red, two pulses administered by 1 ms apart, whereas in blue a 3-ms ISI was applied. The lag of the 3-ms ISI is evident up to 250 ms following stimulus onset. In (j), we quantified the initial response by examining the difference (1 ms vs 3 ms ISI) between the rectified signals. Within both the 5 to 6 ms (t-test;P<0.005;n=13) and the 6 to 7 ms bin (t-test;P<0.05;n=13), a 1-ms ISI led to significantly larger responses than the 3-ms ISI. (k,l) Flat maps with BOLD responses mapped and the recording electrode positions based on the stereotaxic coordinates and mapped unto monkey atlas D99 brain. (m,n) 3D surface rendering with stereotactic grid overlaid (5 mm spacing of grid). DCN stimulation side is indicated with STIM. Figure 5: LFP and BOLD responses following stimulation of the cerebellar output. ( a–h ) LFPs following a 4-pulse burst are shown. Stimulation periods in a–j are indicated by grey rectangles. Sites from which the recordings was obtained are plotted in k and l onto flatmaps for the two monkeys (A05, I04). ( a ) contralateral precentral gyrus (mapped to F1); ( b ) contralateral postcentral gyrus (mapped to 1-2); ( c ) contralateral postcentral gyrus (mapped to 1-2 bordering BA5); ( d ) contralateral precentral gyrus (mapped to F4); ( e ) contralateral postcentral gyrus (mapped to border of 7b and 7op); ( f ) contralateral intraparital sulcus (mapped to AIP); ( g ) ipsilateral intraparital sulcus (mapped to border AIP/7t/7a); ( h ) prefrontal cortex (mapped to BA 46d). A number of traces show high-frequency responses following the stimulus. Contralateral recording sites show greatest deflections at 5–12 ms, with the earliest appearing 2–4 ms ( a–f ). Ipsilateral responses show greatest immediate responses at 5–7 ms ( g ). ( i , j ) DCN stimulation with double pulses. In I, results are shown from recording site G (ipsilateral to DCN stimulation side, mapped to border AIP/7t/7a). In red, two pulses administered by 1 ms apart, whereas in blue a 3-ms ISI was applied. The lag of the 3-ms ISI is evident up to 250 ms following stimulus onset. In ( j ), we quantified the initial response by examining the difference (1 ms vs 3 ms ISI) between the rectified signals. Within both the 5 to 6 ms ( t -test; P <0.005; n =13) and the 6 to 7 ms bin ( t -test; P <0.05; n =13), a 1-ms ISI led to significantly larger responses than the 3-ms ISI. ( k , l ) Flat maps with BOLD responses mapped and the recording electrode positions based on the stereotaxic coordinates and mapped unto monkey atlas D99 brain. ( m , n ) 3D surface rendering with stereotactic grid overlaid (5 mm spacing of grid). DCN stimulation side is indicated with STIM. Full size image We also tested whether the prolonged stimulation was underlying the multifocal pattern. In our usual stimulation protocol, we applied successive pulses for a 200-ms period; therefore, we also tested shorter 10-ms stimulation periods. Pulses delivered at 600 Hz for 10 ms and repeated every 100 ms ( Fig. 4d–f ) gave very similar multifocal activation patterns. Systematic variation of the pulse delivery period (pulse train on) showed that 7 pulses in 10 ms were sufficient to achieve significant BOLD responses ( Fig. 4e ). Purkinje cells are known to inhibit the DCN. One explanation could therefore be that DCN require a higher stimulation frequency to overcome Purkinje cell inhibition. However, directly stimulating the DCN axons by placing the electrode at the SCP—thereby evading Purkinje cell inhibition—yielded similar frequency preferences ( Supplementary Fig. S7 ; 3 SDU reached with 400 Hz and above). Hence another explanation becomes more likely, namely that the shifted saturation of the BOLD responses to higher stimulation frequencies is owing to the fact that the evoked synaptic events are generally small and are still capable of temporally summating at these frequencies. Neurophysiology of cerebello–cerebral responses To achieve a better temporal resolution of the neuronal responses by electrical stimulation of the DCN, we carried out electrophysiological recordings from a number of cortical areas in two monkeys. Direct measurement of neuronal activity was also important in determining whether the BOLD responses observed were due to neuronal activity or to cardiovascular vasopressure responses, as already described previously for stimulating the anterior part of the fastigial nucleus [30] . We observed that the application of a single stimulation pulse led to a fast response in LFP within the contralateral primary motor cortex (stimulation of NIA/SCP in monkey A05; Supplementary Fig. S9 ) although there were no major BOLD responses within areas of the prefrontal cortex ( Supplementary Fig. S10 ). The response appeared within 2–4 ms from the stimulation onset. This would correspond to a conduction velocity of about 20–40 mm ms −1 (assuming a 1 ms synaptic delay and a DCN to cerebral cortex distance of 45 mm). Identical latencies have been recorded in the cat (2–4 ms by ref. 31 ). Figure 5a–h shows the results of administering four pulses within 4 ms. We observed accumulated responses in seven of the areas tested (F1, F4, 3a-b, 1-2, 7op, 7t, AIP). These rapid stimuli were often discernible as summating high-frequency responses (4 in 7 ms=approx. 600 Hz), almost identical to the maximal frequency responses observed in the BOLD signal. To further examine the efficiency of high-frequency stimulation in the DCN output network, we applied paired-pulse stimulation at different intervals. A decline in response amplitude for the shorter intervals would signify the refractiveness of spike generation, whereas an increase for shorter intervals would suggest the presence of a system with fast responses and a short refractory period [32] . We applied successive double pulses, separated by either a 1-ms period or a 3-ms period (inter-stimulus interval (ISI)). Figure 5i shows such an example (obtained from recording site Fig. 5g ). The 1-ms ISI protocol gave rise to a larger short-latency response ( Fig. 5j ). We quantified the initial response by observing the rectified LFP amplitude in the time period of 5 to 6 ms from the stimulation onset. Figure 5j depicts the difference between the two ISI, with the shorter interval showing the larger summated LFP. A quantification demonstrated that these differences were statistically significant ( t -test; P <0.005; n =13). These results show that the pathway has a millisecond temporal summation window. The ability of the pathway to veridically reflect time intervals in the order of a few milliseconds is also indicated by the fact that increasing ISI separation between the 2 pulses by 2 ms resulted in a shift of the early LFP components by exactly the same amount ( Fig. 5i ). The results from the LFP recording experiments are therefore in line with the multisite BOLD responses and support the notion of a temporally highly precise pathway. Temporally highly precise or high-frequency networks have been unravelled in other brain regions such as the motor cortex [33] , the somatosensory cortex [34] and the hippocampus [35] . In contrast to our study, however, these networks, previously implicated in temporally high-precision processing include cerebral cortex only, did not include subcortical components. The fact that high temporal precision is a crucial aspect of cerebellar processing is not entirely unexpected. Indeed, a number of elements in the cerebellum are uniquely adapted to operate in a fast and precise temporal regime. These include special fast potassium and sodium channels that lead to extremely short action potentials of 180 us [36] . Accordingly, high-frequency firing is observed in a number of neurons in the cerebellum [27] , [37] , [38] . DCN firing has been shown to be modulated up to around 100 Hz on average [39] , with some studies reporting maximal frequencies of 450 (ref. 40 ) and 700 (ref. 38 ). These ultrahigh frequencies may be required for the control of fast and very brief movements such as encountered in the oculomotor system [28] and can be understood as a property of the system reflecting its high temporal precision. One intriguing connection comes to mind between the cerebello–cerebral networks' preference for high temporal precision and the uniqueness of the cerebellar–cortical microcircuitry. The most numerous neurons in the cerebellum (in the whole brain, to be precise [8] ) are the granule cells that provide a short-lived excitatory feed-forward computation of the order of milliseconds by their parallel fibres [9] . Hence, any computations occurring within this temporal window require the system to be responsive in the millisecond range. Our neurophysiological results indicate that even a short-lived (~4 ms) burst of stimulation is sufficient to markedly influence a neocortical region. Interestingly enough, well-synchronized pauses in Purkinje cell firing of the order of 15–20ms have been reported to occur in neighbouring Purkinje cells taken as reflections of precise temporal coding in the cerebellum [41] , [42] . If any computations are to occur within this temporal window, the system is expected to show precise responses in the millisecond range. Recent work on the cerebellum has made a convincing case for the cerebellum serving as the substrate of forward models that represent predictions of the sensory consequences of motor acts [43] , [44] , [45] . Continuously updated predictions of the sensory consequences of a movement help to improve motor control by compensating the inevitably long delays of sensory feedback [3] . Moreover, it is indispensable for the precise perceptual separation of sensory stimulation arising from the world from the one resulting from the subject´s activities [46] . Probably the best understood biological realization of this principle is the brainstem saccade generator that relies on an extremely precise and instantaneous prediction of actual eye position rather than on way to sluggish sensory feedback [47] , [48] . Importantly, this internal prediction of the eye movement is optimized by the cerebellum [49] . It is intriguing to note that the regions in motor, parieto-occipital and sensory cortex that were shown to be activated using es-fMRI of the DCN share a common need for sensory prediction input. For instance, area 8 Av, the frontal eye fields [18] , integrates a sensory prediction, in this work usually referred to as corollary discharge or efference copy, to update the target for a second saccade by taking information on the retinal consequences of a first saccade into account. By the same token, monkey visual motion processing area VPS (visual posterior sylvian area) (corresponding to area 7 op in the atlas [23] ) is assumed to take a prediction of the visual consequences of smooth pursuit eye movements into account to generate a veridical percept of motion in the world [50] . Visual motion area (PIVC), most probably the human counterpart of monkey area VPS, has also been implicated in using sensory prediction as well as to acquire this information from the posterolateral cerebellum [51] . These examples, illustrating the role of precise and continuously updated sensory predictions, make it clear that the demonstration of fast and precise cerebellar input to large parts of sensory and motor regions of cerebral cortex is in full accordance with the assumed role of the cerebellum in optimal sensory prediction. We were surprised to find that stimulation of the DCN revealed no major BOLD responses within areas of the prefrontal cortex ( Supplementary Fig. S10 ), some of which are believed to maintain strong connections with the dentate nucleus based on the transsynaptic transport of a rabies virus tracer [24] . The only conceivable explanation we can think of is that we may have missed hitting the fibre bundle in the SCP destined for prefrontal cortex. A final note relates to the striking difference between the rather limited extent of stimulation effects observed after electrical stimulation of striate and extrastriate neocortex, confined to structures receiving monosynaptic input from the stimulation site [10] , [11] , [52] and the widespread polysynaptic stimulation effects seen after stimulating the DCN. Differences in inhibition probably constitute a crucial factor. Stimulation of the neocortex revealed the presence of strong inhibition, thus preventing the propagation of electrically induced activation over multi-synaptic pathways. This is in good agreement with the prominence of inhibition both in its duration [10] , [53] and in the presence of a wealth of different inhibitory interneurons in the neocortex [54] . Comparable inhibitory mechanisms do not seem to matter in the case of stimulation of the cerebellar output. The DCN are, of course, also under prominent inhibitory control by the cerebellar cortex. However, in our experiments, this source of inhibition was bypassed by stimulating DCN axons directly. Surgical and anaesthesia procedures This study involved 22 combined microstimulation-fMRI experimental sessions in four (A06, A07, A05, I04) healthy anaesthetized monkeys (Macaca mulatta) weighing between 4 and 8 kg. The studies were approved by the local authorities (Regierungspraesidium) and were in full compliance with the guidelines of the European Community (EUVD 86/609/EEC) for the care and use of laboratory animals. Recording chambers were centred on the DCN and head holders were custom-made from MR-compatible plastic (PEEK, poly ether ether ketone) and positioned stereo-tactically based on high-resolution magnetic resonance anatomical images. Surgical procedures for implantation of recording chambers and head holders and the anaesthesia protocol during fMRI imaging have already been described [55] . Briefly, the animal was intubated after induction with fentanyl (31 μg kg −1 ), thiopental (5 mg kg −1 ) and succinylcholine chloride (3 mg kg −1 ), and the anaesthesia throughout the experiment was maintained with remifentanil (0.5–2 μg kg −1 min −1 ). Remifentanil is the standard μ-opioid that has been used throughout our previous monkey fMRI experiments [10] , [11] , [21] because of a number of beneficial features at these concentrations: little effect on cerebral metabolism, negligible effects on neuronal excitability (as measured with motor-evoked potentials) and potential neuroprotective effects [56] . In our previous microstimulation fMRI experiments [10] , a comparison between the anaesthetized and awake state did not reveal any substantial differences in evoked BOLD responses. After induction of the anaesthesia, mivacurium chloride (5–7 mg kg −1 h −1 ) was used to assure complete paralysis of the animal to avoid any brain activation induced by muscle contractions (for example, small eye or body movements) during microstimulation. Throughout the experiment, lactate Ringer's with 2.5% glucose was infused at 10 ml kg −1 h −1 and the temperature was maintained at 38–39 °C. Microstimulation of the DCN Recording and microstimulation hardware, including electrodes and microdrives, were mostly developed in-house. A plastic chamber (18 mm inner diameter), formed to fit the animal's skull precisely, was stereotactically implanted during an aseptic surgical procedure and the skull bone inside the chamber was removed. The electrode was inserted into the brain through a fibre glass guide tube with a ceramic tip that penetrated the dura. The electrodes were designed and custom-built using 100 μm (diameter) pure iridium wire, which was bevelled and glass-coated. The glass-coated end of the electrode had a length of 7 mm and was continued with a 45-mm long glass tube of 0.6 mm diameter that, in turn, was glued into a 2-mm glass tube. This ending part fit into a custom-made concentric bronze alloy electrode holder which has also been described previously [55] . The electrode holder was held firmly in a plastic microdrive attached to the recording chamber. The electrode impedances ranged from 40–220 kOhm at the beginning of the experiments and typically reached 30–50 kOhm after microstimulation. The positioning of the electrode was accomplished by manually turning a screw with a thread pitch of 500 μm. The electrode was advanced and the amplified neural signal recorded. Once the electrode penetrated the tentorium and neural activation from the cerebellar cortex was observed, a short anatomical scan (FLASH, echo time(TE)/repetition time (TR)=10/1500 ms, Field of view (FOV)=96×96 mm 2 , 384×256 matrix) in the sagittal plane served as a guide for the precise electrode position and planning of the final electrode positioning to the desired location. For microstimulation, we used a custom-built stabilized current source. Details of the microstimulation hardware set-up are given by Tolias, et al . [11] The current amplitude, pulse duration, train duration and stimulation frequency were controlled digitally using our own TCL-based software and a QNX (Canada)-based real-time operating system. The microstimulation pulse trains consisted of biphasic charge-balanced pulses with the following standard parameters: pulse duration of 200 μs, frequency of 400 Hz, current peak amplitude of 250 μA, pulse trains 200 ms on and 400 ms off. Some parameters, such as frequency, were changed systematically and are indicated appropriately. The microstimulation paradigm started with a 9-s resting period followed by 6 s stimulation and 15 s of resting (in some cases we used 6 s–6 s–18 s). This sequence was repeated between 15 and 20 times during one MRI scan. In our standard electrical stimulation experiments, the ground electrode was composed of a large surface low-impedance connection to the animal consisting of ~10-cm long silver-wire wrapped around gauze soaked in saline and placed in the cheek pouches. We tested the influence of the ground electrode position by replacing it with a different ground electrode positioned diametrically at the dorsal posterior part of the skull (chamber location) and found no differences in the results. During the experiments, the stimulating electrode tip position was verified within the cerebellar cortex and was advanced to the DCN under guidance by high-resolution MRI scans and the neurophysiological LFP/multiunit signal. In one monkey, we reconstructed electrode location by comparing MRI and injecting BDA and obtaining histological sections ( Supplementary Figs S2A, B, E, and F ). The locations of the other electrode were obtained by aligning the high-resolution MR electrode location on the template (A06) of the histologically verified MR (see Supplementary Fig. S1 for further details). MRI data collection Experiments were conducted in a vertical 4.7 Tesla scanner with a 40-cm diameter bore (Biospec 47/40v, Bruker Medical, Ettlingen, Germany). The system had a 50mT m −1 (180 μs rise time) actively shielded gradient coil (BGA 26, Bruker) of 26 cm inner diameter. We used a custom chair and custom system for positioning the monkey within the magnet [55] . Customized radiofrequency volume quadrature coils were used to image the whole brain of the animal. We selected 20 or 22 slices of 2 mm thickness so as to cover most of the macaque's brain. BOLD activity from these slices was acquired at a temporal resolution of 3 seconds per volume with two-shot GE-recalled EPI images (TR/TE=1500/15ms, bandwidth=100kHz, flip angle (FA)=60°, FOV=96 mm×96 mm, Matrix=96×96 reconstructed to 128x128, EPI module duration 51.5 ms). T1-weighted, high-resolution (192×192, reconstructed to 256×256, 0.5 mm thickness) anatomical scans were obtained using the 3D-MDEFT (modified driven equilibrium Fourier transform [57] ) pulse sequence, with an TE of 4.5 ms, TR of 20 ms, FA of 20 deg, and 4 segments. DCN were localized before chamber and/or electrode positioning by acquiring MR images typically with a RARE sequence (rapid acquisition with relaxation enhancement) with a TR of 3500 ms, a RARE factor of 8, effective TE 80–100 ms, 4 averages, FOV=96×96 mm, matrix=256×256 and a slice thickness of 1 mm ( Supplementary Figs S2A and B ). MRI data analysis MRI data were analysed using software developed in MATLAB, as described in detail previously [10] . Preprocessing included spatial smoothing by applying a Gaussian filter (kernel size 3×3, s.d.=1.2; FWHM=2.6 mm). Time courses for individual voxels were extracted, preprocessed by linear detrending and normalized to standard deviation units. Statistical maps were generated using the general linear model (GLM [58] ) with a time-shifted (3 s) box-car model as predictor, by subsequent thresholding at P <0.005 (uncorrected for multiple comparisons) and by applying a clustering algorithm to eliminate random spuriously activated voxels. Clustering was performed by centring a 4×4 window (that is, a window containing 7^2=49 voxels) on each of the activated voxels. Voxel activity was considered spurious if there were not at least another 15 activated voxels within this window. Mapping fMRI responses Two methods were used to map microstimulation-evoked fMRI responses. In the first approach, we mapped neocortical responses on a flat map of a template monkey (D99) with different cortical areas delineated based on the combined MRI and histology atlas of the macaque brain [23] . To this end, we used different routines supplied with the MATLAB package mrVISTA [59] . Basically, for each session, in-plane high-resolution anatomies were aligned and interpolated to the high-resolution anatomy of atlas monkey D99. Alignment was carried out manually by marking about 20 fiducial points on 4–6 corresponding horizontal sections. In a second approach ( Supplementary Figs S5 and S6 ), we mapped subcortical responses within the thalamic nuclei and the brain stem to identify regions that consistently showed good responses. Neurophysiological data acquisition and analysis To verify the nature of the DCN stimulation responses in the neocortex, we combined esfMRI with subsequent neurophysiological recordings in a number of potential neocortical regions. In two monkeys, stimulating electrodes were placed under MR-control within the cerebellar nuclei output tract, that is, the SCP (two white circles in Supplementary Fig. S2E ). Reconstructed electrode position for A051r1/51: AP, 4.75 mm; DV, +9 mm; ML, 3.4 mm and for I043O2/40, electrode position was IAL, AP, 1.8 mm; DV, +7 mm; ML, 2.5 mm. Recording was performed with tungsten-insulated (FHC) electrodes with an initial impedance of 1 MOhm (within-brain impedance of about 130 kOhm at 23 kHz sampling). Neural signals were amplified and filtered into a band of 1–8 kHz (Alpha Omega Engineering, Nazareth, Israel) and then digitized at 21 kHz with 16-bit resolution (National Instruments, Austin, TX, USA), to ensure adequate resolution of local field activities. Electrodes were inserted using a steel guide tube and positions were verified with a KNOPF stereotaxic frame. Electrical stimulation was carried out with bursts at 1 Hz with pulse duration of 200us, amplitude current of 250 μA. Bursts consisted of 4 biphasic pulses within a 4-ms window. For each site, 175 repetitions were acquired. How to cite this article: Sultan F. et al . Unravelling cerebellar pathways with high temporal precision targeting motor and extensive sensory and parietal networks. Nat. Commun. 3:924 doi: 10.1038/ncomms1912 (2012).